Single yeast cells vary in transcription activity not in delay time after a metabolic shift Individual cells respond very differently to changes in environmental conditions. Stochasticity causes cells to respond at different times, magnitudes or both. Here we disentangle and quantify these two sources of heterogeneity. We track the adaptation dynamics of single Saccharomyces cerevisiae cells exposed to a nutrient shift from methionine to sulphate and back. Using single-molecule RNA fluorescence in situ hybridization, we count the number of transcripts of a methionine-biosynthesis enzyme in single cells during adaptation. The variation of response times between cells is small, yet we find a high transient variability in the messenger RNA copy numbers. Surprisingly, single cells display strongly delayed transcription induction, as we could induce transcription fourfold quicker by direct activation and bypassing the cellular control circuitry. Transcription repression occurs rapidly within several minutes. This study indicates that small variability in response timing combined with high, stochastic transcription activity can cause large cell-to-cell variability in dynamic adaptation responses. A period of reduced growth rate, a so-called lag phase, after a nutrient shift is a common phenomenon in microbiology; a famous example is the glucose–lactose diauxie of Escherichia coli , discovered by Monod and coworkers [1] . The general interpretation is that a lag phase results from the time that it takes for the microorganism to adapt its metabolism. Several single-cell studies indicate that the cause for the lag phase can also involve stochasticity: either only a small fraction of the population grows under the new condition [2] , [3] , [4] , [5] , [6] , and the lag phase derives from the time that it takes until those cells reach a significant fraction of the total population; or cells start to grow only after a fluctuation in gene-expression activity has occurred that is large enough to kick-start the induction of the nutrient uptake pathway [7] , [8] , [9] . In both these cases, the lag phases of individual cells vary greatly. The fact that many different adaptation mechanisms can occur may explain the great variation in lag phase durations that have been experimentally observed, which range from minutes to days [2] , [3] , [4] , [7] , [8] . Large variability in response times can occur when cells cannot sense the environmental change, as they lack dedicated sensors. Then they have to rely on stochasticity-induced adaptation mechanisms. This applies for instance to E. coli with respect to lactose and for S. cerevisiae in the case of galactose [4] , [7] , [8] , [9] . In such a case, the organism has to rely on leaky gene expression of dedicated permeases. Alternatively, cells sense the nutrient change and subsequently adjust metabolism without having to resort to stochastic adaptation mechanisms [10] , [11] . Even in this case, stochasticity still plays a role. The inherent stochasticity of molecular reactions and cell growth [12] , [13] , [14] , [15] can still cause cell-to-cell variation in the lag phase of single cells. It is at present much less understood how variable the responses of individual cells are when they are confronted with a condition shift that they can sense. In this work, we study the response of single cells to a shift in their sulphur source from methionine to sulphate and back. This nutrient shift has the advantage that yeast exploits various signalling mechanisms for amino-acid sensing and the initiation of adaptive responses [16] , [17] . This system is therefore ideally suited to answer the question how variable single cells are in their response time (lag phase) when they actively monitor their environment for changes and do not rely on spontaneous stochasticity-induced adaptation mechanisms. Sulphate uptake and assimilation in S. cerevisiae is mainly regulated by the transcriptional activator Met4 [18] , [19] , [20] ( Supplementary Fig. 1 ). In the presence of a high-quality sulphur source, such as cysteine, methionine or S-adenosylmethionine (SAM), Met4 is ubiquitinated by the SCF (Skp1-Cullin-F-box)/Met30 complex. Depending on media conditions, this either targets Met4 for degradation by the proteasome or inhibits its activity as a transcriptional regulator of a set of genes, including the MET genes [21] , [22] . One of those MET genes is MET5 , which encodes the beta subunit of a sulphite reductase required for growth on sulphate to synthesize methionine and related amino acids. The recognition of Met4 as a substrate of the ubiquitin ligase depends on the presence of intracellular cysteine (or a related metabolite) placing the expression of methionine and cysteine biosynthetic genes under negative-feedback control [23] . In the absence of a high-quality sulphur source, Met4 activates the transcription of sulphur uptake, glutathione (GSH) and SAM biosynthesis genes. Among the activated genes is also Met30, which introduces a second negative-feedback loop. Interestingly, cadmium can be used to bypass this complex regulation. It causes dissociation of the SCF (Skp1-Cullin-F-box) ubiquitin ligase and the substrate recognition protein Met30, thereby inhibiting the ubiquitination of Met4 and activating de-ubiquitination of the existing Met4-ubiquitin [24] , [25] . Thus, cadmium allows for the direct induction of gene expression by effectively bypassing the cellular decision process. We use cadmium for this purpose to determine the contribution of cellular decision making to the adaptation delay of single cells. We exploit single-molecule fluorescence in situ hybridization (smFISH) [26] to monitor the dynamics of transcription induction and repression of MET5 in single cells. The advantage of smFISH is that it allows for counting of the exact number of transcript molecules per cell. Most importantly, it allows for exact monitoring of transcription repression. Since the lifetime of fluorescent reporter proteins is typically not the same as the protein it is reporting, the applicability of fluorescent reporter proteins to study transcription repression is limited. Single-molecule RNA FISH has been applied to yeast before to address a wide variety of transcription and cell-to-cell heterogeneity-related questions [27] , [28] , [29] , [30] , [31] , [32] , [33] , [34] . Our results demonstrate that the regulatory systems responsible for metabolite sensing and transcriptional control of the metabolic enzymes can operate very similarly in individual cells, leading to precise timing of the induction of adaptation responses. However, cell-to-cell variability in adaptation dynamics can still be significant. The explanation is that the little variation in response times combined with a steep increase in transcriptional activity causes large differences in transcript copy numbers between cells during their adaption dynamics. Therefore, cell-to-cell variation in response timing and magnitude cooperatively cause large heterogeneity in cellular adaptation dynamics. Nutrient downshift causes a 40-min lag phase in growth We subjected S. cerevisiae to a nutrient downshift from a defined medium containing methionine, and sulphate to the same medium without methionine. With downshift, we mean a change from a preferred nutrient (methionine) to a nutrient (sulphate) that reduces growth rate. 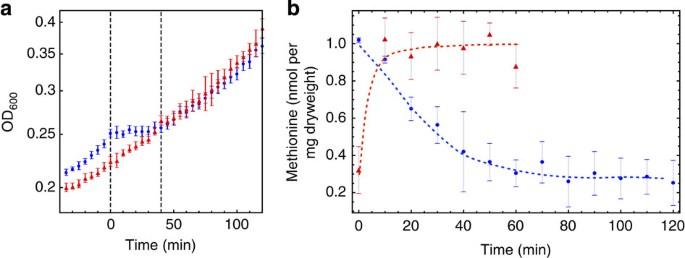Figure 1: Physiological response of a population of yeast cells. (a) Changes in OD600before and after the change in medium at time zero (average±s.d.). Blue circles denote the induction time course (nutrient downshift), red triangles the repression time course (nutrient upshift). (b) Changes in intracellular methionine concentration after the change in medium (average±s.e.m.). Trend lines were added to guide the eye. Concentrations in nmol per mg dry weight can be converted to mM by a conversion factor of ≈0.2 assuming a cell volume of 70 μm3and dry weight of 15 pg per cell. Figure 1a (blue markers) indicates that, at the level of the cell population a lag phase of about 40 min occurs in cell growth. During this period, the intracellular methionine concentration ( Fig. 1b ) decreases very slowly. After 40 min, cells resume growth on sulphate at a slightly lower rate. The intracellular methionine concentration remains at a lower level ( Fig. 1b ). The growth rate drops by about 12% when the cells shift from methionine to sulphate growth, indicating the preference of yeast for methionine. The duration of the generation times on methionine (2.1 h) and sulphate (2.5 h) indicates that the lag phase is much shorter than the generation time. Figure 1: Physiological response of a population of yeast cells. ( a ) Changes in OD 600 before and after the change in medium at time zero (average±s.d.). Blue circles denote the induction time course (nutrient downshift), red triangles the repression time course (nutrient upshift). ( b ) Changes in intracellular methionine concentration after the change in medium (average±s.e.m.). Trend lines were added to guide the eye. Concentrations in nmol per mg dry weight can be converted to mM by a conversion factor of ≈0.2 assuming a cell volume of 70 μm 3 and dry weight of 15 pg per cell. Full size image The fact that growth stops immediately upon the switch to medium without methionine ( Fig. 1a , blue line), that is, before the intracellular methionine concentration depletes significantly, could hint at growth control via extracellular signalling of amino acids [35] , [36] . The intracellular methionine concentrations during the nutrient downshift decreases from 1 to 0.3 nmol per mg dry weight. This reduction is not enough to sustain measurable growth as the sulphur requirement of yeast is ≈90 nmol per mg dry weight [37] , indicating rapid sulphur limitation. Even if GSH reserves, with GSH concentrations about 10-fold higher than methionine concentrations [38] , [39] , would be used as a sulphur source this would not lead to significant growth. So, cells need to activate the sulphate assimilation pathway to synthesize methionine before they can continue growing. They take about 40 min to do so, which is long in comparison with the durations of messenger RNA (mRNA) and protein synthesis; we estimate that synthesis of the first protein takes about 2 min and the steady-state rate depends on the promoter and ribosome-binding site strength, but several transcription initiations per minute have been found experimentally ( http://bionumbers.hms.harvard.edu ). In the complementary nutrient upshift experiment (sulphate to methionine and sulphate), no lag phase is observed ( Fig. 1 ; red markers) and the intracellular methionine concentration returns to its higher value in <10 min. Methionine can be taken up by several specific and non-specific amino-acid transporters [40] , [41] , [42] that are already expressed, which likely explains the quick rise in intracellular methionine concentration after the nutrient upshift. Single-molecule mRNA FISH shows that all cells respond We used smFISH to measure the single-cell dynamics of the MET5 mRNA during the transitions described in the previous section. MET5 encodes the β-subunit of sulphite reductase required for synthesis of methionine during sulphate growth. Cells were fixed at different time points after the medium change, and the MET5 mRNA copy numbers per cell were determined for each time point for on average 1,170 cells per time point ( Fig. 2 ). 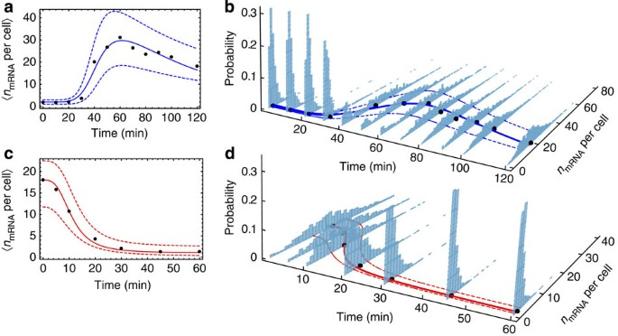Figure 2: Dynamics of the probability distributions of mRNA copy numbers per cell. The induction time course (nutrient downshift) is shown inaandb, and the repression time course (nutrient upshift) incandd. Inaandc, the dynamics of the average copy number per cell, ‹nmRNAper cell›, is shown. Inbandd, the probability distribution for the mRNA copy number per cell is shown as function of time. Ina–d, black dots denote the measured average copy numbers, the solid lines indicate the trend lines for average copy numbers per cell and the dashed lines the 25 and 75% quantiles. For each time point, 800–1,500 cells were analysed. Figure 2: Dynamics of the probability distributions of mRNA copy numbers per cell. The induction time course (nutrient downshift) is shown in a and b , and the repression time course (nutrient upshift) in c and d . In a and c , the dynamics of the average copy number per cell, ‹ n mRNA per cell›, is shown. In b and d , the probability distribution for the mRNA copy number per cell is shown as function of time. In a – d , black dots denote the measured average copy numbers, the solid lines indicate the trend lines for average copy numbers per cell and the dashed lines the 25 and 75% quantiles. For each time point, 800–1,500 cells were analysed. Full size image The distributions for the induction time course ( Fig. 2b ; nutrient downshift) show transient bimodality at the 40–60 min time points, indicating that some cells respond later than others (also shown in Fig. 3b ). We note that the final distributions for both time courses are unimodal. The overlap between the initial and final distribution is small for both time courses, indicating that those states are nearly identical. 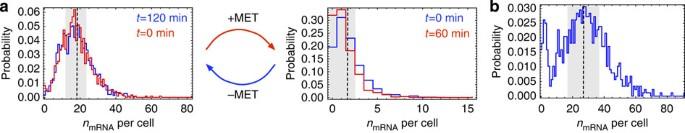Figure 3: Probability distributions indicate reversibility of nutrient shift and transient subpopulations. (a) The steady-state distributions of the upshift (blue) and downshift (red) experiments overlap, indicating the reversibility of this shift. Dashed lines indicate the average number of mRNAs per cell, the shaded area the 50% quantile. (b) During the nutrient downshift, distributions of mRNA copy numbers per cell become transiently bimodal, indicating that some cells respond earlier than others. The distribution of the downshift experiment at the 50-min time point is shown. Figure 3a indicates that cells without any transcripts exist. However, this does not mean that those cells have not responded in the past, as it cannot be ruled out that they have and also experienced significant transcript degradation. In the following sections we will show that all cells do respond to the nutrient shift, using a deconvolution analysis of the dynamics of transcript distributions. Figure 3: Probability distributions indicate reversibility of nutrient shift and transient subpopulations. ( a ) The steady-state distributions of the upshift (blue) and downshift (red) experiments overlap, indicating the reversibility of this shift. Dashed lines indicate the average number of mRNAs per cell, the shaded area the 50% quantile. ( b ) During the nutrient downshift, distributions of mRNA copy numbers per cell become transiently bimodal, indicating that some cells respond earlier than others. The distribution of the downshift experiment at the 50-min time point is shown. Full size image The lag phase observed in the growth profile during the nutrient downshift ( Fig. 1 ; blue markers) is also observed in the transcriptional response: during the first 30 min after induction, the average mRNA copy number per cell increases only slightly, followed by a sharp rise between 30 and 50 min. We speculate that the two negative-feedback loops, occurring in the gene network controlling MET5 transcription (see Introduction and Supplementary Fig. 1 ), are responsible for the overshoot observed in the mRNA copy numbers per cell observed during the nutrient downshift experiment. As these feedback loops involve transcriptional regulation, they occur on a slower timescale than the metabolic system that they control and therefore constitute delayed negative feedbacks. The nutrient upshift experiment ( Fig. 2c,d ) indicates hardly any delay in transcription repression Fig. 2b . In Fig. 3a , we illustrate the reversibility of nutrient shift as the start and the end state of nutrient shift experiments are nearly identical. Figure 3c shows the transient bimodality of the probability distribution for MET5 transcripts during the induction experiment. Thus, at time point 50 min the population consists of two subpopulations, those cells that have responded and those that have not yet done so. Large cell-to-cell variation during induction and repression Figure 2 indicates significant cell-to-cell variability in the response to the nutrient up- and downshift. We characterize the magnitude of the cell-to-cell variability in the mRNA number per cell in Fig. 4 with the fano factor, as well as the correlation between the copy numbers in the nucleus and the cytoplasm. The fano factor is defined as the copy-number variance divided by the mean copy number. A fano factor equal to one corresponds to a simple model, where mRNA is synthesized by a zero-order reaction and degraded by a first-order reaction [43] . Fano factors higher than one can indicate temporal fluctuations in the synthesis rate, either through transcriptional bursting or due to noise in the concentrations of molecules that influence transcription rate such as, for instance, RNA polymerases and transcription factors [44] . We note that the use of the fano factor is most informative when applied to unimodal distributions; hence, its application at time points 35–70 min is an approximation. However, already at time 50 min most probability mass lies around the higher transcript levels. 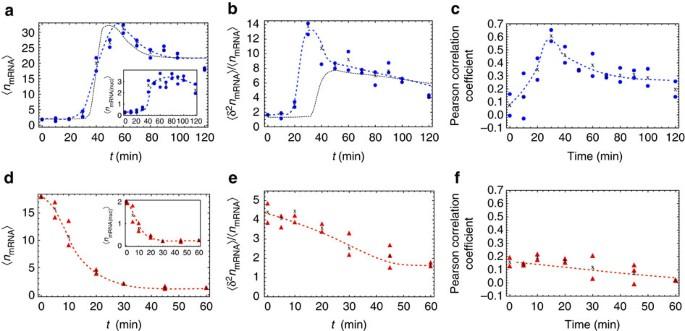Figure 4: Peaks in the fano factor and correlation profiles in the induction time courses indicate a delay in transcription induction. (a,d): averages of the numbers of transcripts per cell (insets show the numbers per nucleus). (b,e): fano factors of numbers of transcripts per cell. (c,f): Pearson correlation coefficient between the number of RNA molecules in the nucleus and in the cytoplasm during the time courses. The upper plots correspond to the induction time course, and the lower row of plots to the repression time course. Coloured markers (circles, triangles) denote results of individual experiments, black markers the results for the pooled data. Trend lines (coloured) were added to guide the eye. The black dashed lines inaandbindicate the profiles that would be obtained if all cells started induction at the exact same time. Note that the scale of the axes differs between the time courses. Figure 4: Peaks in the fano factor and correlation profiles in the induction time courses indicate a delay in transcription induction. ( a , d ): averages of the numbers of transcripts per cell (insets show the numbers per nucleus). ( b , e ): fano factors of numbers of transcripts per cell. ( c , f ): Pearson correlation coefficient between the number of RNA molecules in the nucleus and in the cytoplasm during the time courses. The upper plots correspond to the induction time course, and the lower row of plots to the repression time course. Coloured markers (circles, triangles) denote results of individual experiments, black markers the results for the pooled data. Trend lines (coloured) were added to guide the eye. The black dashed lines in a and b indicate the profiles that would be obtained if all cells started induction at the exact same time. Note that the scale of the axes differs between the time courses. Full size image Fluctuations in transcription activity lead also to positive correlations between mRNA numbers in the nucleus and the cytoplasm. This can be understood intuitively in the regime of fluctuations that are slow in comparison with the rate of export to the cytoplasm and the rate of transcript degradation. In this regime, the copy numbers in the nucleus and in the cytoplasm reach a quasi steady state before the synthesis rate changes significantly. While the synthesis rate is higher than its time-averaged value, both quasi steady-state averages are also higher than their time-averaged values (and vice versa for a synthesis rate below its time average), leading to a positive correlation between the transcript numbers in the nucleus and the cytoplasm. Experimentally observed correlations are shown in Fig. 4c,f . The magnitude of the correlation depends on the timescale and magnitude of the fluctuation and the shape of its autocorrelation function, as well as the rate of mRNA export from the nucleus and the lifetime of transcripts (see Supplementary Fig. 2 for an illustration). All experimentally observed correlations are positive or zero. In contrast, variations in the rate of nuclear export would lead to a negative correlation. Again, this can be understood intuitively since high export rates lead to transiently lower than average transcript numbers in the nucleus and higher than average numbers in the cytoplasm. Variations in the rate of RNA degradation (in the cytoplasm) by themselves do not introduce correlations between numbers in the nucleus and the cytoplasm: they reduce the magnitude of correlations introduced by other mechanisms ( Supplementary Fig. 2 ) (assuming that the degradation rate fluctuations are independent of fluctuations in synthesis and/or export). Copy number per cell is positively correlated with volume, therefore some of the correlation could be explained if also the cytoplasmic and nuclear volume are positively correlated, which is expected for a population in balanced growth. When a subset of cells with defined volume is considered instead of the whole population, the magnitudes of the correlations do indeed decrease by ~30% but the profile remains the same ( Supplementary Fig. 3 ). For both experiments, we observe fano factors >1 during all time points ( Fig. 4b,e ). The correlations between mRNA numbers in the nucleus and the cytoplasm are positive throughout the up- and downshift experiment. At the steady states, the fano factor of the transcript copy number distribution, as well as the correlation between the numbers of mRNA in the nucleus and in the cytoplasm are higher in the induced state than in the repressed state ( Fig. 4d,e ). This indicates that either the magnitude of the extrinsic fluctuations is higher during the induced state or that the timescale of these fluctuations relative to the lifetime of mRNA is slower in the induced than in the repressed state. The nutrient upshift experiment can be used to estimate the half-life of the mRNA. By fitting a delayed exponential decay to the average number of mRNA per cell over time in this experiment ( Supplementary Fig. 4 ), we calculate a half-life of about 7 min, that is, much shorter than one generation time. Previously, values between 13 and 18 min were reported for the half-life of MET5 mRNA [45] , [46] , [47] ). Therefore, the intrinsic fluctuations in transcript levels can be expected to have a corresponding autocorrelation time, such that such fluctuations in mRNA persist with a characteristic lifetime of about 7 min. Assuming that the protein lives much longer and, therefore, responds in level at much slower timescales, we expect that the intrinsic fluctuations in mRNA have no influence on protein levels and on metabolic flux. However, the fano factor of transcripts indicated the occurrence of extrinsic noise, for instance from promoter switching, and this can occur on timescales close to the protein lifetime. Hence, we cannot exclude from this data that the extrinsic noise in mRNA propagates to protein and causes fluctuations in enzyme activity. Homogeneous time delay in transcription induction To assess the delay times in transcription responses, we determined at each time point the fraction of cells that has not yet (transcriptionally) responded. The method we used is described in detail in Supplementary Note 1 . Briefly, we assume that the copy-number distribution at a given time point after the nutrient shift is the convolution of the steady-state distribution before the shift, and the distribution for the net new synthesis (nutrient downshift) or degradation (nutrient upshift) of transcripts. The fraction of cells that have not (yet) responded to the nutrient shift at that time point then corresponds to the probability for a net new synthesis/degradation of zero transcripts. This assumes that the number of newly synthesized molecules does not depend on the number of molecules that a cell has at time zero. Since molecule numbers depend on volume, we repeated this analysis for subsets of cells with similar volumes ( Supplementary Fig. 5 ). The result obtained with this approach did not change the conclusions of this section. From the change in the fraction of cells that have not yet responded over time, we can deduce the response time distribution ( Fig. 5 ; method explained in Supplementary Fig. 6 ). 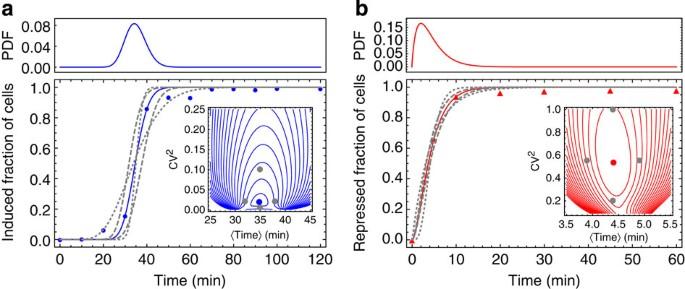Figure 5: The RNA FISH distribution of the induction time course fits only a peaked delay time distribution. The change in the fraction of induced or repressed cells over time (a: nutrient downshift,b: nutrient upshift) is shown along with the cumulative density function (CDF) of a gamma-distributed delay time. The coloured line corresponds to the best fit, the grey lines to nearby parameter combinations (inset). The probability distribution of the best fit is shown above each plot. The insets show contour plots of the fitting objective (the mean squared error) as a function of the average delay time and its squared coefficient of variation along with dots marking the best fit (blue, red) and the parameter combinations that are shown in the main figure (grey). Note that the scale of the axes differs between the time courses. Figure 5: The RNA FISH distribution of the induction time course fits only a peaked delay time distribution. The change in the fraction of induced or repressed cells over time ( a : nutrient downshift, b : nutrient upshift) is shown along with the cumulative density function (CDF) of a gamma-distributed delay time. The coloured line corresponds to the best fit, the grey lines to nearby parameter combinations (inset). The probability distribution of the best fit is shown above each plot. The insets show contour plots of the fitting objective (the mean squared error) as a function of the average delay time and its squared coefficient of variation along with dots marking the best fit (blue, red) and the parameter combinations that are shown in the main figure (grey). Note that the scale of the axes differs between the time courses. Full size image For the nutrient downshift the, delay times can only be fitted with peaked distributions ( Fig. 5a ). The shape of the delay time distribution for the nutrient upshift was not well constrained by the data and could be fitted by either exponential or peaked (gamma) distributions ( Fig. 5b ). Remarkably, the nutrient downshift is fitted best with delay time distributions with a very small coefficient of variation (<0.1), indicating that the response time is very homogenous across the cell population. Different peaked distributions (gamma, normal and lognormal) fit the data equally well. Direct determination of the transcription rate from the data gave similar average delay times ( Supplementary Note 2 ; Supplementary Fig. 7 ). In Supplementary Note 3 and Supplementary Figs 8 and 9 , we show that part of the delay time heterogeneity during the nutrient upshift can be explained by a dependence of the delay time on the cell volume at the time of nutrient shift. To assess to what extent the heterogeneity in the delay time causes cell-to-cell variability in the response, we calculated the time profiles of the average copy and its variance that would be obtained if there was no delay time heterogeneity (described in Supplementary Note 4 ). The fano factor profile obtained in this way for the nutrient downshift experiment ( Fig. 4b , dashed line) is no longer peaked and shows a monotonous increase from the repressed to the induced state. This suggests that the small heterogeneity in the delay time is sufficient to cause the peaked fano-factor profile observed in the experimental data. An analogous analysis could also be applied to the correlations between nuclear and cytoplasmic mRNA copy numbers, but did not yield insightful results due to error propagation. Next, we calculated from the data the exact contribution of delay time variability and response magnitude variability to variability in the adaptive response of the cells. To achieve this, we decompose the cell-to-cell variability, as quantified by the copy-number variance, at each time point into one part caused by the heterogeneity in delay times and another that captures stochastic mRNA synthesis and degradation: Fig. 6 shows this decomposition for the nutrient downshift experiment. While the population consists of a mixture of cells that already have induced transcription and cells that have not, the variance is dominated strongly by the contribution deriving from delay time heterogeneity. This is mainly caused by the steep rise in mRNA copy numbers upon induction, so that small differences in response time cause large differences in the expected copy number at individual time points. But due to the small delay time heterogeneity (CV<0.1), this regime only lasts for ≈15–20 min after which the variance contributions from transcript synthesis and degradation become dominant again. 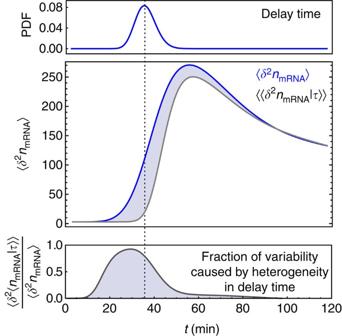Figure 6: Delay time heterogeneity is transiently the dominant cause for copy-number variation during the nutrient downshift. Total variance in mRNA copy numbers for the nutrient downshift experiment (‹δ2nmRNA›; blue line) and variance due to sources other than the delay time variability (‹δ2nmRNA|τ›; grey line). The difference between these two variances is shown as the grey shaded area and equals the variance contribution of the delay time heterogeneity. The bottom panel shows the fractional contribution of the delay time variability. The best fit delay time distribution is depicted in the top panel. The vertical dashed line marks the average delay time. Figure 6: Delay time heterogeneity is transiently the dominant cause for copy-number variation during the nutrient downshift. Total variance in mRNA copy numbers for the nutrient downshift experiment (‹ δ 2 n mRNA ›; blue line) and variance due to sources other than the delay time variability (‹ δ 2 n mRNA | τ ›; grey line). The difference between these two variances is shown as the grey shaded area and equals the variance contribution of the delay time heterogeneity. The bottom panel shows the fractional contribution of the delay time variability. The best fit delay time distribution is depicted in the top panel. The vertical dashed line marks the average delay time. Full size image Direct transcription activation reduces delay time fourfold The delay time of about 35 min for induction of gene expression ( Fig. 2 ) and resumption of growth ( Fig. 1 ) appears long, given that mRNA and protein synthesis times are expected to be of the order of a few minutes. To test whether cells can initiate transcription faster and that the delay is due to delayed induction of gene expression by pre-transcription control mechanisms, we performed a time course experiment using cadmium to induce transcription of the MET genes. Cadmium is a known strong and direct activator of the sulphate assimilation pathway [24] , [25] . We added cadmium to the medium with methionine and sulphate. The induction of MET5 transcription after addition of cadmium chloride displays a delay of about 8 min, which is considerably shorter than the transcription induction after the nutrient downshift ( Fig. 7 ). This shows that cells can activate transcription much faster than the delay time of 40 min observed during the nutrient downshift. Supplementary Figure 10A indicates that cell growth slows down more and more over time until it stops after about 100 min, presumably due to the toxic effects of cadmium. We therefore only consider the cadmium response up to a time point of 45 min. Supplementary Figures 10–13 illustrate that the qualitative stochastic properties of the delay time distribution and transcription stochasticity are preserved when cadmium is added. The intracellular methionine concentration ( Supplementary Fig. 10B ) decreases in a manner very similar to the nutrient downshift experiment (although the medium still contains high concentrations of methionine). A similar decrease has been observed previously by Lafaye et al. [39] and is likely explained by a shift in the pools of sulphur-containing metabolites after cadmium treatment to increase the GSH concentration. 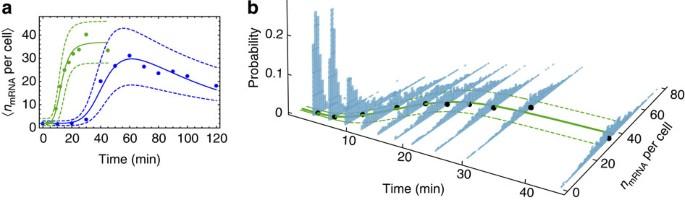Figure 7: Cadmium reduces the delay time for transcription induction of MET5. (a) The solid lines indicate the average copy number per cell (green: cadmium addition, blue: nutrient downshift; as inFig. 2), and the dashed lines the 25 and 75% quantiles. (b) mRNA copy-number distributions for the cadmium addition experiment at different time points. Figure 7: Cadmium reduces the delay time for transcription induction of MET5. ( a ) The solid lines indicate the average copy number per cell (green: cadmium addition, blue: nutrient downshift; as in Fig. 2 ), and the dashed lines the 25 and 75% quantiles. ( b ) mRNA copy-number distributions for the cadmium addition experiment at different time points. Full size image Unicellular organisms have to adapt to environmental changes to sustain fitness and thereby prevent being out-competed by other species. They do so by adjusting their metabolic machinery upon nutrient changes. We studied the single-cell response of yeast to a shift in their sulphate source. The interpretation of our findings is that, since S. cerevisiae can attain a higher growth rate on methionine than on sulphate, it ‘prefers’ methionine when growing on both sulphur sources ( Fig. 1 ). When suddenly confronted with a lack of methionine (a nutrient downshift) it has to adjust its metabolism causing a growth delay ( Fig. 1 ). Only after an unexpectedly long delay of about 35 min does yeast induce the expression of the methionine synthesis pathway ( Fig. 2 ) that feeds on sulphate. When from this condition confronted with methionine addition (nutrient upshift), yeast immediately assimilates it and stops transcription of the methionine synthesis pathway ( Fig. 2 ). These findings are in agreement with earlier findings on sulphur-source shifts with yeast [48] , [49] , [50] . Earlier studies on different nutrient shifts have reported the existence of a subpopulation of cells that does not respond at all [2] , [3] , [5] , [6] or the occurrence of very dispersed response times [4] , [7] , [8] across a range of microbial species. In these cases, stochasticity in the cell population is large, mostly due to stochasticity in response times, leading either to a bimodal or very broad distribution of cell responses. In contrast, we find that all yeast cells responded (to the up- and downshift) with remarkably similar response times for transcription induction ( Fig. 2 ). These findings agree with the fact that S. cerevisiae uses a dedicated signalling network to sense methionine absence and subsequently induce transcription of the MET genes [16] , [17] . The existing studies that have reported widely dispersed response times, that is, for the gal regulon in S. cerevisiae [4] and the lac operon in E. coli [2] , [7] , [8] , are all cases where nutrient signalling is absent. The case that we report here is more similar to the study of Muzzey et al. [51] on the hyperosmotic shock response of single yeast cells where also all cells responded quickly and a dedicated sensing network is involved. Our study therefore indicates that we should distinguish between single-cell responses to environmental (including nutrient) changes that involve active sensing mechanisms and those that lack sensing mechanisms. Although we found that the single yeast cells induced a response at almost the same time, the subsequent transient transcription activity proved very heterogenous between cells ( Figs 2 , 3 , 4 ). Whereas in the existing studies [2] , [3] , [4] , [5] , [6] , [7] , [8] the cellular heterogeneity is mostly due to large variability in response times, we find appreciable cellular variability due to differences in response magnitude at low response-time variability. The small coefficient of variation for the response-time distribution for the nutrient downshift experiment (CV 2 ≈0.02) is characteristic for a very accurate induction time of a process. Nonetheless, this little delay time heterogeneity is transiently the dominant source of copy-number variations ( Fig. 6 ). This is caused by the strong increase in mRNA copy numbers (≈20-fold), such that even small differences in timing between cells lead to large transient copy-number variations. Summarizing, a cell that is induced a little earlier in time than another already has produced several transcripts, hereby causing the appreciable transcript noise ( Fig. 6 ). The mechanism of noise generation that we report in this study derives from the number of transcripts that can be produced during a characteristic timescale for delay time variability. So, if transcription activity is high then during the time that corresponds to one delay time s.d., a significant amount of transcripts can be made even when this s.d. is small, causing significant (transient) cell-to-cell variability. For instance, if the transcription activity, υ , is deterministic and equals 10 transcripts per minute and the s.d. in the delay time, σ τ is either 1 min or 30 s, then in the 1-min case the s.d. in the number of transcripts, σ n , will be highest (expected to be proportional to υ · σ τ because ). Additional noise in transcription activity will increase the variability in transcript numbers even more. This type of noise-generating mechanism is very similar to transcription bursts where also a timescale and an activity together give rise to burst statistics [52] . Whereas insightful measures exist for noise of steady-state systems, such as the coefficient of variation and bimodality, measures for characterization of variability in transient responses of cells are much less standardized. In this work, we took a simple view and reasoned that cells can have very variable dynamic responses through three mechanisms. In the case of response-magnitude variability, cells have a deterministic response time and a stochastic activity. During response-time variability, cells have a deterministic activity and stochastic response time. The last case is that response-magnitude and response-time variability mix. The experimental study described in this work is an example of the last mode, but with a firm bias towards response-magnitude variability. This work indicated how high activity and little delay time variance can still cause a significant variation in single-cell transcript dynamics. We think that this simple classification is very useful for the comparison of other systems. Most of the experimental cases published so far are response-time variability systems, because these cases are biased to systems without active sensing mechanisms. The two cases that we are aware of that involve sensing systems (ours and ref. 51 ) are both examples of dominating magnitude variability. Our data indicate that all cells eventually adapt to the down- and upshift experiment. In case of the upshift experiment, methionine likely enters the cell via unspecific amino-acid transporters [16] , [17] and is immediately metabolized by the active metabolic network ( Fig. 1 ) presumably leading to a transcription repression signal. In the downshift experiment, all cells eventually induced gene expression indicating that they all sensed the methionine removal and the presence of sulphate. Although invariable fluctuations in signalling components of the amino-acid-sensing network will occur, they are apparently not impeding the ability of single cells to identify the nutrient shift and induce an adaptive response. Similar conclusions were drawn for the osmoregulation control system in yeast [51] . This indicates that cellular decision making can be very robust to inevitable noise in its molecular components. Although we did find very stochastic transcription activity, this is likely not propagated to the metabolic activity and fitness. As long as mRNA fluctuations occur on a fast enough timescale such that they do not propagate to protein levels, protein function, which contributes to fitness, is not compromised and natural selection will likely not punish fluctuations in mRNA levels. This we expect to be very common, as the timescales of transcription bursting [12] and the lifetimes of mRNAs [53] are typically much shorter than the response time of metabolic enzymes, which tend to have characteristic times close to the generation time [14] , [53] . Our cadmium induction experiments indicate that the delay time in transcription induction upon methionine removal is due to processes preceding transcription regulation. Why yeast cells do not respond in this quick mode in the nutrient downshift is not entirely clear. It is unlikely that the molecular events preceding transcription, that is, sensing and subsequent transcription factor activation, take over 30 min. So, it is tempting to conclude from this that yeast cells are delaying the decision to induce the methionine synthesis pathway. Presumably because this is such a costly pathway to make, they anticipate that methionine may return soon and have sufficient sulphur storage to survive for about 30 min. By waiting they do not waste valuable resources on enzyme synthesis of the methionine biosynthesis pathway—for which they do not get a return of investment if methionine reappears and as a consequence they suffer a loss of fitness. This would either suggest that yeast has evolved in a fluctuating methionine environment with a characteristic time of methionine shortages of about 30 min, or for some other reason its storage capacity is only sufficient to delay the decision to induce the costly pathway by 30 min. In addition to methionine storage capacity, the regulatory roles of methionine and SAM can also contribute to the observed transcription response delay. Reduction of the intracellular methionine level is perceived by yeast and initiates several stress response mechanisms, such as a growth stop and, eventually, autophagy [54] , [55] . However, methionine has a particularly complicated role in cell survival and growth control [56] . The origin of the delay upon methionine removal may therefore also be related to a general growth rate and stress-related signalling mechanism. The molecular details of this global response are currently subject to active research [54] , [55] . It will be interesting to see whether other nutrient shifts of single cells that involve sensing mechanisms display delayed decision making, and how this relates to nutrient storage and the evolutionary history of those organisms. We predict that the response systems that do not involve sensing mechanisms operate in a much more stochastic regime, as has already been found for the glucose–lactose shift in E. coli where adaptation is primarily induced stochastically [7] , [8] . In these latter cases, the stochasticity in response timing and magnitude add up, which may cause large cell-to-cell variability over extended time periods. When active environment sensing occurs, heterogeneity in transcription delay time can be greatly reduced, but still its contribution to cell-to-cell copy-number variability can be large when transcription activity is high. Strains and growth conditions S. cerevisiae strain YSBN6 (MATa, FY3 ho::HphMX4) was used for all experiments. Cells were grown in synthetic medium [57] at a pH equal to 5, supplemented with 2% glucose at 30 °C, 200 r.p.m. For all experiments, cells were first cultured on a plate, inoculated into a small volume of medium and grown into exponential phase. From this culture, a larger volume was inoculated and grown to OD 600 =0.25–0.3 when the time courses were started. For the repression time, course cells were cultured in medium without any addition (but from a medium containing sulphate) and the time course started by addition of 20 mg l −1 L -methionine (final concentration). For the induction and cadmium time courses, cells were cultured in medium supplemented with 20 mg l −1 L -methionine, and at time zero either shifted to a medium without methionine or CdCl 2 was added to a final concentration of 0.5 mM. Determination of intracellular methionine levels Cells were grown up to OD 600 =0.25–0.3 and time courses were started by addition of L -methionine (20 mg l −1 final concentration) or cadmium (0.5 mM final concentration) or shifting the cells from a medium with 20 mg l −1 methionine to a medium without methionine, and samples were taken every 10 min. Intracellular metabolites were extracted as described by Canelas et al. [58] , with quenching in −40 °C methanol and extraction using the boiling ethanol method. Dry weight was determined in 60-min intervals. Samples were labelled with O -phthaldialdehyde (Sigma P0657) and amino-acid concentrations were determined on a Shimadzu HPLC with a C18 Agilent ZORBAX Eclipse plus C18, Solvent saver plus 3.0 × 150 mm 3.5-micron column. Norvalene was used as the internal HPLC standard to correct for differences in labelling efficiency from sample to sample. The column was equilibrated in 98% buffer A (5 mM sodium azide, 10 mM sodium tetraborate, 10 mM Na 2 HPO 4 , pH 8.2), 2% buffer B (45% methanol/45% acetonitrile/10% H 2 O, (v/v/v)) and the concentration of buffer B was increased to 57% over a time of 30 min with a flow rate of 0.64 ml min −1 . Single-molecule mRNA FISH Single-molecule mRNA FISH was performed as described by Raj et al. [59] with modifications: Cells were grown up to OD 600 =0.25–0.3 and fixated with formaldehyde (final concentration 3.7%) first for 40 min at room temperature, then continued overnight at 4 °C. After two washes with buffer B (1.2 M sorbitol, 0.1 M potassium phosphate, pH 7.5), spheroplasting was performed with 25 μg lyticase (Sigma L2524) in buffer B in a total volume of 250 μl at 37 °C. Progression of spheroplasting was monitored using phase-contrast microscopy, and spheroplasting was continued until approximately half of the cells appeared as phase-dark. Cells were washed twice with buffer B and the cell pellet was stored overnight in 70% ethanol. Samples were hybridized with a final probe concentration of 1.5 nM in hybridization buffer (2 × saline-sodium citrate (SSC), 10% formamide (v/v), 10% dextran sulphate (w/v), 1 mg ml −1 transfer RNA, 2 mM vanadyl ribonucleoside complex and 0.2 mg ml −1 bovine serum albumin) at 37 °C. Cells were washed twice with 2 × SSC/10% formamide with 30-min incubations at 37 °C in between. 4′,6-diamidino-2-phenylindole (DAPI) was added in the first wash step after hybridization. 3′-amine-modified DNA oligos (Biosearch Technologies, Novato, CA) were labelled with NHS-ATTO565 (ATTO-TEC GmbH, Siegen, Germany) by dissolving 1 nmol of each oligo in 50 μl 0.1 M sodium bicarbonate solution, adding 200 μg of dye and incubating at room temperature for 1 h in the dark. Oligos were concentrated by ethanol precipitation and HPLC purified on a C18 column using a gradient of 7–30% acetonitrile and 93–70% 0.1 M triethyl ammonium acetate, pH 6.5, over a course of 30 min with a flow rate of 1 ml min −1 . Oligonucleotide sequences are listed in Supplementary Table 1 . Image acquisition Samples were mounted in 2 × SSC and imaged using a Nikon Ti-E scanning laser confocal inverted microscope, CFI Plan Apo VC × 60 oil objective and Nikon NIS-Elements AR imaging software. A 561.5-nm diode-pumped solid state and 402.1 nm diode lasers were used for excitation; detection was via 595–50 nm and 450–50 nm bandpass filters. Optical sections were captured at 0.250-μm intervals and a pixel size of 0.1243 μm in lateral dimensions, resulting in a voxel size of 0.0039 μm 3 . Four times averaging was used to reduce photon and camera noise. Image analysis Images from the ATTO565 channel were background corrected using a two-dimensional (2D) median filter of radius 5 pixels (where the median filtered image was used as an estimate for the background image). An initial spot identification was performed based on binarizing a LoG-filtered image as described by Raj et al. [26] with automated thresholding as in Itzkovitz et al. [60] : the s.d. divided by the mean calculated over a window of length 7 of the number of spots versus threshold function was maximized yielding the threshold where the spot number is least dependent on the exact choice of threshold. Since the density of spots was very high for some of the conditions, in these binary images many regions correspond to multiple single-molecule mRNA spots. This can also be seen in the curves of spot counts versus the threshold for binarization ( Supplementary Fig. 14 ): for low spot densities the spot count decreases monotonically with increasing threshold, while for high spot densities the curve goes through a minimum followed by a maximum before spot counts finally decrease to zero. This is because while higher thresholds will lead to the exclusion of some true spots, higher thresholds will also split large regions that correspond to multiple spots that are close together. The automated thresholding will in those cases find the local maximum as the threshold, which would lead to the exclusion of some low-intensity spots that would be included in a low spot density image. Therefore for all images that had a spot count versus threshold profile with a local minimum followed by a local maximum, the initial threshold was then shifted to the local minimum. For all images, large regions that had multiple local intensity maxima were subdivided until all regions had a size in accordance with a single diffraction-limited spot. Segmentation of nuclei was performed based on the DAPI image using a global threshold that maximizes the total number of nuclei within the correct size range. The maxprojection of the nuclei segmentation image along the z axis was used as a marker image for a watershed segmentation on a z-section of the transmitted light image to determine the cell outlines in 2D. Regions that fell outside of a specified size range were rejected. Outlines were inspected and cells that the automatic segmentation procedure had missed were added manually. Cells were subsequently segmented in three-dimensional based on the cell background fluorescence in the DAPI channel. A global threshold was determined using Otsu's method (minimization of intraclass variance) after excluding the grey values from regions identified as nuclei. The three-dimensional outline of a cell was taken as the region in the binary image that fell within the 2D outline determined previously. Statistical tests on RNA FISH data All experiments were performed at least as duplicates; the cell numbers for each time point from cumulated experiments is >800 for all time points. To test for the reliability of the spot-finding procedure, the distributions of copy numbers per cell for each individual image (most images contain between 20 and 50 cells) were compared with the accumulated distribution from all other images from the same experiment by a Pearson χ 2 -test. After correction for multiple testing, only one image gave a significant P -value; manual inspection of the spots found in this image did not indicate an obvious malfunction of the spot-finding procedure. For each experiment many images were acquired consecutively. Owing to the long imaging times with confocal microscopy, some slides were under the microscope (at room temperature) for several hours. When plotting the average copy number per cell for each image normalized to the total average versus the order the images were acquired, no bias was observed towards lower spot counts in later images ( Supplementary Fig. 15 ). Volumes of cells and nuclei were both estimated from the signal in the DAPI channel. Owing to the small size of these volumes in comparison with the pixel dimensions, those measurements have a relatively large relative error. In addition, the time for which cells were kept in ethanol before hybridization varies between experiments, which could also lead to differences in the cell volumes. Supplementary Figure 16 shows the distributions of cell and nuclear volumes. There is no indication for a change in the volume distributions over the time course of the experiments (see inset of Supplementary Fig. 16 ), but the averages for single experiments differ by up to 15% from the total average. Therefore all analyses are performed by comparing the smallest/intermediate/largest third of the cells. How to cite this article: Schwabe, A. et al. Single yeast cells vary in transcription activity not in delay time after a metabolic shift. Nat. Commun. 5:4798 doi: 10.1038/ncomms5798 (2014).